High-speed panoramic light-sheet microscopy reveals global endodermal cell dynamics The ever-increasing speed and resolution of modern microscopes make the storage and post-processing of images challenging and prevent thorough statistical analyses in developmental biology. Here, instead of deploying massive storage and computing power, we exploit the spherical geometry of zebrafish embryos by computing a radial maximum intensity projection in real time with a 240-fold reduction in data rate. In our four-lens selective plane illumination microscope (SPIM) setup the development of multiple embryos is recorded in parallel and a map of all labelled cells is obtained for each embryo in <10 s. In these panoramic projections, cell segmentation and flow analysis reveal characteristic migration patterns and global tissue remodelling in the early endoderm. Merging data from many samples uncover stereotypic patterns that are fundamental to endoderm development in every embryo. We demonstrate that processing and compressing raw image data in real time is not only efficient but indispensable for image-based systems biology. Understanding how biological tissues grow and sculpt organs of varied size, shape and function is one of the most intriguing questions in developmental biology today [1] . Non-invasive fluorescence microscopy is the primary tool to observe, track and quantify the development of biological specimens, but the imaging of living vertebrate embryos has been a challenge due to their size and opacity. Recently, light-sheet microscopy [2] , [3] , such as selective plane illumination microscopy (SPIM) [4] , has been shown to be a valuable technology that performs especially well in samples that are too large for conventional techniques, for example, confocal microscopy. In SPIM, instantaneous optical sectioning is achieved by illuminating the sample with a sheet of light and generating fluorescence in a thin slice, which is then imaged with a fast camera. Millimetre-sized specimens can be reconstructed by rotating and imaging them from different sides (multi-view imaging) [5] . Photo-toxicity in SPIM has been shown to be negligible even at high acquisition rates [2] , [6] . As a result, the imaging speed is becoming less dictated by how much light the sample can tolerate, rather, it is more determined by the camera’s speed. With the development of fast, high-resolution sCMOS cameras, the rate and amount of data generated by SPIM is approximately three orders of magnitude higher than that of conventional confocal microscopes ( Supplementary Fig. S1 ). SPIM setups with one or more sCMOS cameras [7] , [8] , [9] may deliver important new information but at the same time present a major burden of data transfer, storage and management. Therefore, in many high-resolution microscope setups the number of experiments is limited by the available storage, which precludes the rigorous statistical analysis of image data needed for quantitative developmental biology. The issue of long-term storage can be tackled by compression of data [8] ; however, data processing, visualization and analysis are still challenging as the dimensions of the images and the number of voxels do not change. Raw data rates may exceed 1 GB s −1 , though may be far less dense in information content. Consequently, there is a need to process, condense and analyse these data ‘on-the-fly’. One way to efficiently reduce the data stream would be to exploit knowledge about the shape of the sample. Microscope data sets are usually a series of flat images of planar sections and therefore cuboidal, independent of the object’s shape. For flat cell cultures or fixed tissue sections this may not be an issue. Many organisms however exhibit a spherical or ellipsoidal shape, such as embryos of major model organisms (zebrafish, frog, fruit fly and so on), and their cuboidal images are unnecessarily large and offer no dedicated way for visualization. We found that image transformations tailored to the shape of the sample can be performed in real time and efficiently compress the data stream from the microscope. Analysis and visualization of the desired scientific information become straightforward even when many samples are imaged. The endoderm, one of the three germ layers, which is distributed as a monolayer on the surface of the spherical yolk during early stages of zebrafish development, exemplifies that it is essential to image the entire tissue with high spatial and temporal resolution. Whereas most studies on endoderm development have primarily focused on fate specification and organ formation [10] , [11] , little is known about the coordination of cells in space and time that patterns the tissue. Early endoderm migration is of immense importance for organ formation, as defects in cell movement during gastrulation result in duplication or mis-positioning of organs [12] . In the past, the endoderm has been analysed in isolated axial maximum intensity projections of small areas, where the projection is approximately orthogonal to the surface [13] , [14] . These limitations are now overcome in our system: To quantify and understand cell behaviour in gastrula-stage zebrafish embryos, we designed a four-lens SPIM system with integrated real-time image processing that delivers radial maximum intensity projections at high speed. These undistorted high-resolution images of the entire endoderm are computed during the acquisition, in contrast to existing visualization techniques for three-dimensional (3D) data sets of fixed [15] and live [7] Drosophila embryos. In our approach, a typical data set requires Gigabytes instead of Terabytes and offers visualization and evaluation of cell migration in the context of entire embryos right out of the microscope. Taking insights from cartography, two-dimensional (2D) map projections are generated to visualize the entire tissue in a single image. Real-time data registration eliminates any movement of the embryo in its chorion and registers all embryos to a common, predefined coordinate system. Finally, cell tracks are computed to visualize cell localization, density and global migration dynamics in the zebrafish endoderm. We demonstrate that dedicated real-time image transformations efficiently reduce the data stream from the microscope and provide visualizations of complex morphological processes in whole embryos for the systematic analysis of a large sample size. Four-lens SPIM setup for panoramic endoderm imaging Light-sheet microscopy offers a number of advantages over conventional fluorescence microscopy techniques, in particular low photo-toxicity, fast and sensitive detection, and good penetration in scattering tissues [2] , [3] , [4] . Multi-view acquisition makes SPIM the ideal tool for in vivo imaging of millimetre-sized samples, which cannot be imaged entirely from a single side [5] , [16] . Combined with a fast ultrasonic rotational motor, a classical two-lens SPIM setup with one illumination and one detection lens can provide multiple views in a few seconds. Extending this approach, multidirectional SPIM uses a second illumination lens to uniformly excite the focal plane with superior penetration 17 . Furthermore, adding a second detection lens simplifies the acquisition as two opposing views are captured when scanning the sample through the light sheet [7] , [8] , [9] . We built a four-lens SPIM system ( Fig. 1a ) that delivers multiple views at high-speed and is optimized for capturing the entire zebrafish endoderm. 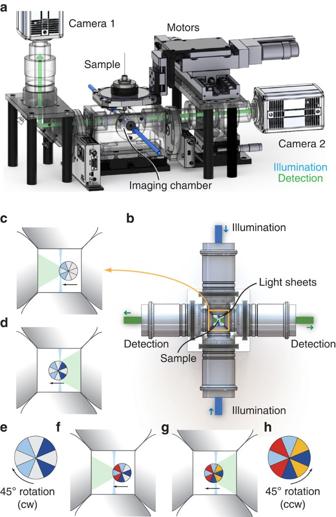Figure 1: Four-lens SPIM setup and image acquisition. (a) Schematic of the central unit of the four-lens SPIM setup. The sample dips into the medium-filled imaging chamber from the top. It is held and moved by a fast rotational stage and three linear motors. Light-sheets illuminate the sample from two opposite sides (blue arrows) and two cameras record the fluorescent signal orthogonally to the light sheets (green arrows). The cameras are precisely aligned to image the same plane. (b) The central imaging chamber consists of four identical lenses for two-sided illumination and two-sided detection of the sample (view from the top). The illumination objectives alternately excite the shared focal plane of the two detection lenses. (c–h) Steps involved in image acquisition. (c) As the sample is moved through the light sheet (arrow), two sectors are well illuminated and detected by the left detection arm (light blue). (d) During the second half of the stack, the right detection arm acquires parts on the right (dark blue). (e) The sample is rotated by 45° and (f,g) complementary regions are imaged in a similar manner (red and yellow), covering the entire sample. (h) The sample is rotated back by 45° and these steps are repeated for time-lapse acquisition (see alsoSupplementary Movie 1). Figure 1: Four-lens SPIM setup and image acquisition. ( a ) Schematic of the central unit of the four-lens SPIM setup. The sample dips into the medium-filled imaging chamber from the top. It is held and moved by a fast rotational stage and three linear motors. Light-sheets illuminate the sample from two opposite sides (blue arrows) and two cameras record the fluorescent signal orthogonally to the light sheets (green arrows). The cameras are precisely aligned to image the same plane. ( b ) The central imaging chamber consists of four identical lenses for two-sided illumination and two-sided detection of the sample (view from the top). The illumination objectives alternately excite the shared focal plane of the two detection lenses. ( c – h ) Steps involved in image acquisition. ( c ) As the sample is moved through the light sheet (arrow), two sectors are well illuminated and detected by the left detection arm (light blue). ( d ) During the second half of the stack, the right detection arm acquires parts on the right (dark blue). ( e ) The sample is rotated by 45° and ( f , g ) complementary regions are imaged in a similar manner (red and yellow), covering the entire sample. ( h ) The sample is rotated back by 45° and these steps are repeated for time-lapse acquisition (see also Supplementary Movie 1 ). Full size image The central unit of our setup consists of four identical objective lenses ( Fig. 1b ). The two detection lenses and their associated optics image the common focal plane onto two sCMOS cameras. A linear stage moves the sample along the detection axis through the focal plane, triggering the acquisition of the cameras every two microns. The two illumination lenses alternately illuminate the focal plane with laser light at every position during the scan. The cameras capture an image of the entire field of view of ~1.2 mm 2 at 62.5 frames per second (f.p.s.). As the cameras had been aligned to provide identical images from two opposing views, no image registration is required to merge the two. Zebrafish embryos (5 h post fertilization (h.p.f.)) were embedded in 1.5% low-melting agarose in an fluorinated ethylene propylene (FEP) tube [6] . To visualize the endoderm, the transgenic zebrafish line Tg(sox17:EGFP) [13] , [18] , which expresses green fluorescent protein in all endodermal cells as well as the dorsal forerunner cells (DFC), was used. The chorion was left intact to provide ideal conditions for the embryo to develop [6] . The tube was mounted onto the stage, dipping into the medium-filled imaging chamber from the top. As the sample was moved through the light sheets, the cameras acquired the well-resolved sectors of the embryo ( Fig. 1c,d ). This process took <10 s. We found that the image quality improved further when the embryo was rotated by 45° with a high-speed ultrasonic piezo motor at each time point to acquire a second, complementary view ( Fig. 1e–h ). A total of eight image stacks (two views for each illumination-detection lens pair) were acquired ( Supplementary Movie 1 ). The additional view improved image quality mainly in the parts of the embryo directly facing the illumination lenses, which were not very well detected due to the larger optical path through the embryo and the limited axial resolution, and in the parts directly facing the detection lenses, which were obliquely illuminated. Owing to the fast motors and the high acquisition rate no developmental changes between the individual views were observed, ensuring that the embryo could be reconstructed in its entirety to visualize the process of endoderm patterning. Real-time processing The shape of an early zebrafish embryo can be approximated by a sphere. On its surface, the endoderm forms a single-cell layer. Projecting the acquired 3D image volume onto the surface of a sphere captures all information about this layer in a single 2D image ( Fig. 2 , Supplementary Movie 2 ). To prepare for a radial projection in real time, a number of steps were performed before each experiment. First, fluorescent beads embedded in agarose were imaged from different angles. The resulting stacks were computationally registered, providing the transformation matrix to align both views ( Supplementary Methods ). Stage drifts were found to be negligible for the typical duration of an experiment. We therefore used the same transformation matrix throughout the time-lapse. 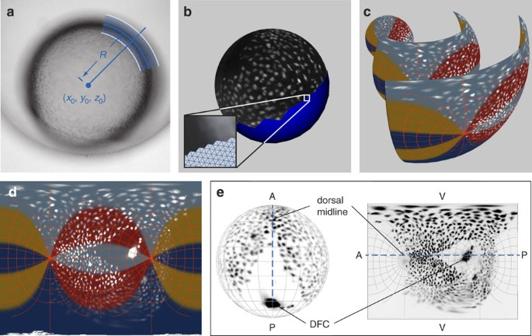Figure 2: Spherical projection and real-time processing. (a) A sphere is fitted to a series of transmission images of a zebrafish embryo. The coordinates of the centre (x0,y0,z0) and the radius (R) are determined. A shell of 140 μm thickness around the sphere surface (blue shaded region) will contribute to the projection. (b) The surface of the sphere is divided into vertices (inset). A ray is cast from the sphere centre to each vertex, and the maximum intensity along each ray within the shell is recorded. (c) The resulting spherical maximum intensity projection is then unwrapped to obtain a 2D map of the spherical data (Supplementary Movie 2). Different colours indicate the parts of the embryo that were recorded by the two cameras from two different angles (compareFig. 1). (d) All endodermal cells spread around the entire embryo are visible in a single image (Supplementary Movie 3). (e) Spatial orientation of the embryo in 3D and on the final map projection. A, anterior; P, posterior; V, ventral; DFC, dorsal forerunner cells. Figure 2: Spherical projection and real-time processing. ( a ) A sphere is fitted to a series of transmission images of a zebrafish embryo. The coordinates of the centre ( x 0 , y 0 , z 0 ) and the radius ( R ) are determined. A shell of 140 μm thickness around the sphere surface (blue shaded region) will contribute to the projection. ( b ) The surface of the sphere is divided into vertices (inset). A ray is cast from the sphere centre to each vertex, and the maximum intensity along each ray within the shell is recorded. ( c ) The resulting spherical maximum intensity projection is then unwrapped to obtain a 2D map of the spherical data ( Supplementary Movie 2 ). Different colours indicate the parts of the embryo that were recorded by the two cameras from two different angles (compare Fig. 1 ). ( d ) All endodermal cells spread around the entire embryo are visible in a single image ( Supplementary Movie 3 ). ( e ) Spatial orientation of the embryo in 3D and on the final map projection. A, anterior; P, posterior; V, ventral; DFC, dorsal forerunner cells. Full size image Transmission light through one of the detection lenses was used to position the embryo in the chamber and to determine the start and end of the stack for both angles. A transmission stack was captured, showing in each plane a different part of the embryo’s surface in focus. A sphere was fitted to these in-focus regions, resembling the surface of the embryo ( Fig. 2a , Supplementary Fig. S2 , Supplementary Methods ). The surface of the sphere was evenly sampled, resulting in a list of ~2.7 million vertices ( Fig. 2b ). Rays were sampled from the centre of the sphere to all vertices. A lookup table was prepared that associated voxels within a shell of 140 μm around the embryo surface with the corresponding vertex index ( Fig. 2a,b , Supplementary Fig. S3 ). For the second view, the fitted sphere was transformed with the known registration matrix before sampling the rays. Eight tables were calculated this way, for each combination of illumination side, camera and acquisition angle. These initial steps to prepare for the time-lapse acquisition took about 10 min. During the actual acquisition, the values of the relevant pixels of every image were assigned to the vertices according to the lookup table. For each vertex, only the maximum value was saved at the end of the stack. At every time point, the eight projections obtained in this way were fused to yield a complete picture of the embryo ( Fig. 2c–e , Supplementary Movie 3 ). We registered the data of consecutive time points to eliminate global movements of the embryo in the chorion such as the turning at the end of gastrulation ( Supplementary Movies 4 and 5 ). Fusion and registration were run in parallel on a separate computer. Our experiments ran for 12 h, one time point every 30 s. Performance analysis using offline data revealed that our radial projection implementation runs with up to 250 f.p.s. and can thus easily keep up with the acquisition speed of the cameras (62.5 f.p.s.). The amount of data was reduced by a factor of ~240 compared to the raw data stream, from 13 TB to 56 GB. Map projections The challenge of visualizing and analysing spherical data has been well studied over decades in the geographical sciences and a number of projections have been developed 19 , each with well-defined properties. We applied several of these projection methods to the spherical data of the zebrafish endoderm ( Fig. 3 , Supplementary Movie 6 ). The conformal (angle-preserving) Mercator projection was calculated parallel to the acquisition as instant visual quality control and later to depict the orientation of cell flow during a time-lapse experiment ( Supplementary Movie 7 ). The area-preserving Bonne and Gall-Peters projections were calculated to quantify the distribution of cell densities. The Winkel Tripel projection gave a good overview of the data with minimal overall distortion. In addition, the raw vertex data was kept for further processing such as cell tracking. 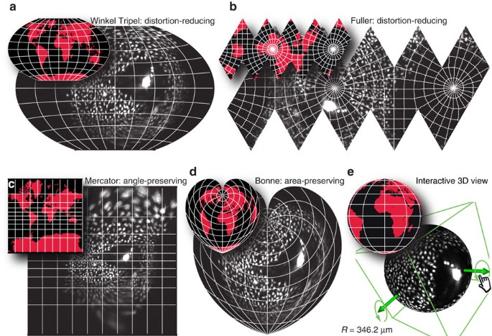Figure 3: Map projections to visualize the entire endoderm. Various map projections are available to quantify different parameters and visualize patterns of cell organization (Supplementary Movie 6). (a,b) Winkel Tripel and Fuller projections show little distortion and are best suited to visualize the speed of cell migration. (c) Angle-preserving Mercator projections were used to visualize cell flows and direction of cell movement. (d) The Bonne projection is area preserving and was therefore used to depict cell densities. (e) Cell dynamics on the spherical data were also visualized interactively in Fiji’s 3D viewer28, where the embryo can be turned to look at specific regions of interest. Insets in the top left corner depict the respective world map projections in red. Figure 3: Map projections to visualize the entire endoderm. Various map projections are available to quantify different parameters and visualize patterns of cell organization ( Supplementary Movie 6 ). ( a , b ) Winkel Tripel and Fuller projections show little distortion and are best suited to visualize the speed of cell migration. ( c ) Angle-preserving Mercator projections were used to visualize cell flows and direction of cell movement. ( d ) The Bonne projection is area preserving and was therefore used to depict cell densities. ( e ) Cell dynamics on the spherical data were also visualized interactively in Fiji’s 3D viewer 28 , where the embryo can be turned to look at specific regions of interest. Insets in the top left corner depict the respective world map projections in red. Full size image Multi-layer projections A single radial projection as described above can be applied to monolayered tissues such as the early endoderm. To make our approach more generally applicable we extended our software to multi-layer projections. The shell around the surface of the sphere, considered for the projections, was now subdivided into thin concentric spherical shells with R i+1 = R i + dR . For each shell the maximum along each ray was computed separately yielding a set of projections, one for each radius R i = R 1 ,..., R N ( Fig. 4a ). The thickness of the shells dR and the number of layers N can be adjusted depending on the morphology of the sample. 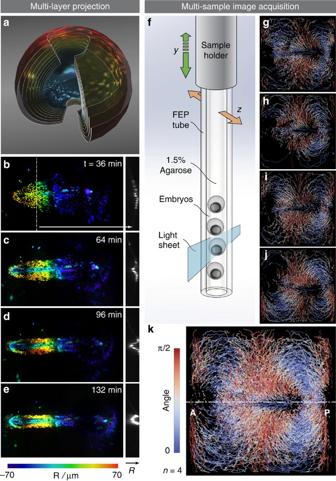Figure 4: Multi-layer projections and multi-sample acquisition. A multi-layer projection is created to capture the radial movement of cells during late gastrulation. (a) Rendering of a radial multi-layer projection, cut open to show the different layers, which are colour coded for different radii. (b–e) Time-lapse multi-layer Mercator projections of a late gastrulation stage embryo. Colour code indicates the radial position of cells from the innermost (blue) across 20 layers to the outermost (red) layer (Supplementary Movie 8). For comparison, cross-sections along the dotted line are shown on the right. (f) Schematic representation of multi-sample data acquisition. Multiple embryos are mounted in agarose in one FEP tube. A motor controls the position alongyand positions each embryo in the light sheet in front of the objective lenses. Projections are then recorded by moving the embryo through the light sheet alongz. (g–j) Four embryos were imaged in parallel (Supplementary Movie 9) and the cell tracks computed. Colour code indicates the unsigned angle between each track and the dorsal midline (dashed line ink). (k) Overlay of the cell tracks fromg–j. Figure 4: Multi-layer projections and multi-sample acquisition. A multi-layer projection is created to capture the radial movement of cells during late gastrulation. ( a ) Rendering of a radial multi-layer projection, cut open to show the different layers, which are colour coded for different radii. ( b – e ) Time-lapse multi-layer Mercator projections of a late gastrulation stage embryo. Colour code indicates the radial position of cells from the innermost (blue) across 20 layers to the outermost (red) layer ( Supplementary Movie 8 ). For comparison, cross-sections along the dotted line are shown on the right. ( f ) Schematic representation of multi-sample data acquisition. Multiple embryos are mounted in agarose in one FEP tube. A motor controls the position along y and positions each embryo in the light sheet in front of the objective lenses. Projections are then recorded by moving the embryo through the light sheet along z . ( g – j ) Four embryos were imaged in parallel ( Supplementary Movie 9 ) and the cell tracks computed. Colour code indicates the unsigned angle between each track and the dorsal midline (dashed line in k ). ( k ) Overlay of the cell tracks from g – j . Full size image In the radial multi-layered projections, the raw 3D data is converted into another 3D representation for the sample, which includes only the relevant parts of the sample in a form that can be easily visualized and analysed. For example, the layers can be colour-coded and overlayed ( Fig. 4b–e ). The multi-layer projections proved to be important at later stages during development when the tissue undergoes invagination at the dorsal midline of the embryo ( Fig. 4d,e , Supplementary Movie 8 ) as well as in recordings where more than just the endoderm is fluorescently labelled ( Supplementary Fig. S4 ). At the same time, the amount of data was still reduced by a factor of ~240/ N . Cell dynamics in the zebrafish endoderm A complete understanding of the molecular and cell biological mechanisms underlying cell dynamics and patterning of the endoderm requires long-term imaging of the entire tissue combined with thorough quantitative analyses. During gastrulation, endoderm cells perform a random walk to rapidly spread on the yolk surface, followed by convergence and extension movements to gather along the embryonic axis [12] , [13] , [14] ( Supplementary Movie 7 ). The chemokine receptor Cxcr4a is expressed in the gastrula-stage endoderm and has been implicated in the regulation of endodermal cell migration. Two previous studies using morpholino-mediated (morphant) knockdown of Cxcr4a function described distinct endodermal phenotypes and proposed very different models for the role of Cxcr4a in endoderm migration. Mizoguchi et al. [13] showed that the Cxcr4a ligand, Cxcl12b, can act as a chemoattractant for endodermal cells, and proposed that Cxcl12/Cxcr4a are required for chemotaxis and dorsal convergence movements of the endoderm [13] . In contrast, Nair and Schilling [12] showed that Cxcr4a is required for transcriptional activation of integrin β1b and endodermal cell adhesion, and proposed a model where Cxcr4a is required for the tethering of endodermal cells to mesoderm in the early gastrula-stage embryo. cxcr4a morphant endodermal cells displayed a marked shift towards the animal pole [12] , a phenotype which was also observed in the cxcr4a s421 mutant ( Supplementary Fig. S5 , unpublished observation by P.A. ), and which might obscure defects in dorsal convergence movements as assessed by in situ hybridization for sox17 (refs 12 , 13 ). To investigate the role of Cxcr4a in controlling endodermal cell migrational behaviour, we used our four-lens SPIM setup to image the entire endoderm in control and cxcr4a morphant Tg(sox17:EGFP) embryos, starting at 6 h.p.f. However, due to the low density of endodermal cells and the inevitable variance in cell location between embryos, a comprehensive map of global tissue flow can only be established by gathering and merging data from multiple samples. Multi-sample acquisitions We adapted our setup so that several embryos can be imaged in parallel. Up to six embryos were embedded in the same tube and one embryo after the other was positioned in front of the objectives using the vertical stage ( Fig. 4f ). This way all samples were imaged sequentially within 1 min and the development of different genotypes, for example, wild-type and cxcr4a morphant embryos, can be directly compared over time. Now an embryo can be reconstructed in its entirety in one of two possible recording modes: For ultimate image quality the embryos are rotated once for a total of eight data stacks as described above. Alternatively, the additional view is omitted to save time and image more embryos in parallel. We recorded the development of four embryos in parallel using the four-lens SPIM setup without rotation ( Supplementary Movie 9 ). To analyse the cellular movements that pattern the endoderm, we segmented the cells ( Supplementary Movie 10 ) and quantified various parameters using the original spherical representation and appropriate map projections. Flow maps were used to depict the path of cells and their angle with respect to the dorsal midline on Mercator projections ( Supplementary Movie 11 ). While each embryo exhibits a slightly different flow pattern ( Fig. 4g–j ), the convergence movement of cells, with their tracks orthogonal to the dorsal midline, is present in all embryos and was visualized by overlaying all the tracks ( Fig. 4k ). Endodermal cell migration in WT and cxcr4a morphants Time-lapse images of wild-type embryos showed cells on both lateral surfaces converging towards the dorsal midline while the embryonic axis extended in the A-P-direction ( Fig. 5a–d , Supplementary Movie 7 ). Anteriorly located cells began to converge during early gastrulation ( Fig. 6a ) and progressed later to more lateral regions ( Fig. 6c ). The laterally located cells migrated in a directed manner, orthogonal to the midline (as seen by the red tracks in Fig. 6a,c , Supplementary Movie 11 ). In contrast, in cxcr4a morphants, the cells failed to converge properly at the midline ( Figs. 5e–h and 6b,d ; Supplementary Fig. S6 and Supplementary Movies 12 and 13 ), consistent with the report of Mizoguchi et al. 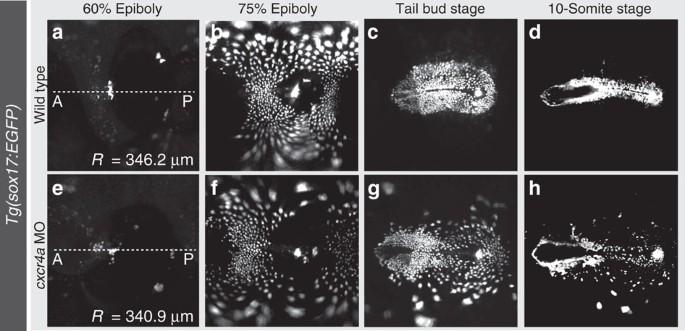Figure 5: Visualizing endoderm cell dynamics in wild-type and crxcr4a morphant embryos. Time-lapse images of the entire developing endoderm in Mercator projections.Tg(sox17:EGFP)line was used to visualize the endoderm from 60% epiboly to 10-somite stage (a–d) in wild type and (e–h) incrxcr4amorphant (Supplementary Movies 7 and 12). The radius of the fitted sphere (R) is stated for the individual data sets. [13] Figure 5: Visualizing endoderm cell dynamics in wild-type and crxcr4a morphant embryos. Time-lapse images of the entire developing endoderm in Mercator projections. Tg(sox17:EGFP) line was used to visualize the endoderm from 60% epiboly to 10-somite stage ( a – d ) in wild type and ( e – h ) in crxcr4a morphant ( Supplementary Movies 7 and 12 ). The radius of the fitted sphere ( R ) is stated for the individual data sets. 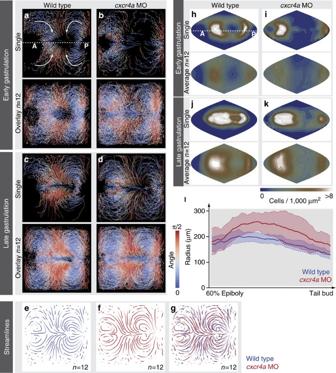Figure 6: Quantification of endoderm cell dynamics reveals conserved flow patterns. For quantitative analysis, movies were split into early (60–75% epiboly) and late gastrulation (75% epiboly, tail bud). (a–d) Orientation of cell migration (a,c) for wild type and (b,d) forcxcr4amorphants calculated on the angle-preserving Mercator projection (Supplementary Movies 11 and 13). Cell tracks from single embryos are shown on the top, the overlay of cell tracks from 12 embryos below. The colour scale indicates the unsigned angle between the cell track and the dorsal midline, direction of cell movement is indicated by white arrows ina. (e,f) Streamlines obtained from the cell tracks of multiple wild-type andcxcr4amorphant embryos to depict the overall flow pattern of endoderm cells during gastrulation. (g) Overlay of streamlines of wild type (blue) andcxcr4amorphants (red,n=12 each). Maps from different embryos were registered with the position of DFCs at tailbud stage for the overlay. (h–k) Spatial distribution of cells as kernel-density estimate on the area-preserving Bonne projections (h,j) for wild type and (i,k) forcxcr4amorphants (Supplementary Movie 14). Cell densities from single embryos are shown on the top, the averaged density distribution from 12 embryos below. The colour scale indicates local cell density from 0 to >8 cells/1,000 μm2. (l) The distance between DFCs and the approaching endoderm margin during the course of gastrulation, obtained by calculating the 0.1 quantile of the cellular distributions in wild type (n=12, blue) andcxcr4amorphant (n=12, red) (Supplementary Fig. S8). The line graph represents the mean distance and the shaded region the standard deviation. In all images the equator corresponds to the dorsal midline, anterior to the left. Full size image Figure 6: Quantification of endoderm cell dynamics reveals conserved flow patterns. For quantitative analysis, movies were split into early (60–75% epiboly) and late gastrulation (75% epiboly, tail bud). ( a – d ) Orientation of cell migration ( a , c ) for wild type and ( b , d ) for cxcr4a morphants calculated on the angle-preserving Mercator projection ( Supplementary Movies 11 and 13 ). Cell tracks from single embryos are shown on the top, the overlay of cell tracks from 12 embryos below. The colour scale indicates the unsigned angle between the cell track and the dorsal midline, direction of cell movement is indicated by white arrows in a . ( e , f ) Streamlines obtained from the cell tracks of multiple wild-type and cxcr4a morphant embryos to depict the overall flow pattern of endoderm cells during gastrulation. ( g ) Overlay of streamlines of wild type (blue) and cxcr4a morphants (red, n =12 each). Maps from different embryos were registered with the position of DFCs at tailbud stage for the overlay. ( h – k ) Spatial distribution of cells as kernel-density estimate on the area-preserving Bonne projections ( h , j ) for wild type and ( i , k ) for cxcr4a morphants ( Supplementary Movie 14 ). Cell densities from single embryos are shown on the top, the averaged density distribution from 12 embryos below. The colour scale indicates local cell density from 0 to >8 cells/1,000 μm 2 . ( l ) The distance between DFCs and the approaching endoderm margin during the course of gastrulation, obtained by calculating the 0.1 quantile of the cellular distributions in wild type ( n =12, blue) and cxcr4a morphant ( n =12, red) ( Supplementary Fig. S8 ). The line graph represents the mean distance and the shaded region the standard deviation. In all images the equator corresponds to the dorsal midline, anterior to the left. Full size image The chemoattractant model predicts that loss of Cxcr4a function should affect the directionality of endodermal cells. To quantify directionality independent of cell distribution, we extracted a general profile of tissue flows by computing the mean orientation of flow through each point in space (averaged across time and samples). The resulting flow fields were visualized with streamlines, indicating the general patterns of cell motion present during gastrulation ( Fig. 6e,f ). We found that the averaged streamlines show a consistent flow pattern, which becomes more complete with increasing sample size ( Supplementary Fig. S7 ). Surprisingly, the streamlines of cxcr4a morphant endodermal cells were indistinguishable from those of wild-type cells ( Fig. 6g ; n =12) indicating that the direction of movement is not affected in the absence of Cxcr4a function. An alternative model is that the early mis-positioning of endodermal cells affects later dorsal convergence movements. To visualize how the spatial distribution of endoderm cells change over time, we calculated cell densities on the area-preserving Bonne projections. The distribution of cells in cxcr4a morphants during early gastrulation appeared more asymmetric with a clear bias towards the anterior side as compared with wild type ( Fig. 6h–k , Supplementary Movie 14 ). Again, to merge data from multiple embryos and reveal common characteristics the density maps were averaged. For a more precise quantification of this asymmetric distribution in a well-defined reference frame, we calculated cell densities in annular regions of increasing radii around the DFCs for each time point ( Supplementary Fig. S8 ). The asymmetry was consistent with the previously observed anterior shift of endoderm cells [12] , resulting in a larger gap between the DFCs and the endoderm margin. In both wild-type and cxcr4a morphant embryos, the mean distance between DFCs and the endoderm margin was found similar at 60% epiboly. However, in cxcr4a morphants this gap increased up to a maximal width of 250 μm (65 μm higher than that in the wild type) before decreasing, further demonstrating the anterior shift of endoderm cells in cxcr4a morphants ( Fig. 6l , n =12 each). The higher variation in the gap sizes of morphant compared with control embryos reflects a higher embryo-to-embryo variability that is commonly seen with morpholino injections. Our analysis shows that loss of Cxcr4a function affects the early distribution and subsequently the end-point position of endodermal cells, without affecting directionality, indicating that the dorsal convergence defects observed in cxcr4a morphant endoderms are due not to a loss of directionality but rather to the relatively longer distance that these cells have to migrate to reach the dorsal midline by the end of gastrulation. These results suggest that Cxcr4a is not required for chemotaxis, and illustrate the requirement for global imaging and multi-sample analysis to understand the true nature of cell migration defects in mutants and morphants such as cxcr4a . We have built a dedicated four-lens SPIM setup providing multiple views at high speed and combined it with a novel, real-time processing engine. In contrast to common 3D imaging approaches, we took advantage of the spherical geometry of the zebrafish embryo to extract the desired information while efficiently reducing the amount of data. The raw data from the cameras were not saved at any point. On the one hand, this means that any additional 3D information that is not captured in the projection gets lost and the projection cannot be repeated at a later time point. On the other hand, the radial projection is an effective compression that immediately delivers preprocessed data for further analysis. Therefore, even though the presented real-time processing will not eliminate the need for slow 3D imaging techniques in more complex shapes, it is a very effective strategy to streamline further analysis and increase throughput in this and other applications. In contrast to axial projections, our radial maximum intensity projection preserved the topology of the tissue. The entire endoderm was imaged quickly with high image quality and displayed for fast visual inspection and precise quantification without distortions irrespective of the actual radius of the sample. The data were conveniently displayed using appropriate map projections, which not only facilitate the analysis of tissue-wide cell movements but also eliminate the potential errors in conventional axial projections. The comprehensive data sets are essential to understand the complex cell behaviours during endoderm development and the dissection of the molecular mechanisms that control these behaviours, such as the chemokine receptor Cxcr4a. Our results suggest that the anterior shift in the endoderm cell distribution in cxcr4a morphant embryos accounts for the defects observed in dorsal convergence during late gastrulation. Imaging an entire tissue with high spatial and temporal resolution may reveal details of developmental processes in the embryo under observation. At the same time, the information from an individual sample needs to be compared to a large ensemble to quantify the variability and the significance of the findings. Therefore, the goal in quantitative developmental biology should be to combine the ideal microscopy technique with appropriate image processing that allows fast visualization and direct analysis of the data. In light sheet microscopy, due to its low photo-toxicity and fast acquisition, data processing has become a serious bottleneck. The presented imaging pipeline gives an example of efficient image acquisition and processing in real time, compromising neither on acquisition speed nor on lateral resolution. Single-cell dynamics and processes at the level of whole tissues can now be simultaneously visualized and correlated. We have combined our multi-sample mounting and acquisition protocols to image many samples in parallel with data processing routines to merge the data from individual embryos, for example, into streamlines or averaged density maps. Further work is now needed to apply this novel toolbox to high-throughput microscope setups to obtain the high sample rates essential for developmental systems biology. The solution presented here is applicable not just for the zebrafish embryo but also for other spherical samples and can be adapted to other convex shapes such as fly embryos, worms and so on. As shown, it can also be extended to multi-layered tissue by replacing the single radial maximum intensity projection with a multi-layered stack. Multi-layer projections can preserve the surface topology and account for, quantify and recover non-spherical samples. Even though our image-processing pipeline runs very efficiently in Fiji 20 on a common workstation computer, the calculations could be performed even faster on dedicated hardware, ideally directly on the frame grabber card or even inside the camera. Instead of storing and post-processing large volumes of image data, the automated extraction of relevant information in real time opens the door for quantification of features in a large number of samples at high speed. SPIM hardware The four-lens SPIM setup consists of four identical water-dipping Olympus UMPLFLN 10x/0.3 objectives, two for illumination and two for detection. The sample chamber was custom-made from acrylic with four openings sealed with rubber o-rings. The sample position and the light sheets are monitored with a webcam through a glass window on the bottom of the chamber. Two Toptica iBeam smart (488 nm, 200 mW) lasers were externally triggered for alternating double-sided illumination. Each beam was guided with an optical fibre onto a continuously running galvanometric mirror (1 kHz, EOPC) for even fluorescence illumination (multidirectional SPIM 17 ). Light sheets were generated with cylindrical lenses and projected with telescopes and the illumination objective lenses onto the common focal plane of both detection lenses. The average excitation power in the entire object plane was ~6 mW per arm. The focal planes of the two detection objectives were imaged onto two Andor Zyla sCMOS cameras through emission filters (Chroma ET BP525/50). Both cameras were precisely aligned via a focusable tube lens and an adjustable mirror to acquire images from the same focal plane, which were streamed to separate computers. The sample was moved and rotated with three motorized linear stages (M-404.1PD/6PD, M-112.1DG) and one rotational stage (M-660.55, Physik Instrumente) using a custom-made software ( Supplementary Methods ). Zebrafish Zebrafish were handled in accordance with EU directive 2011/63/EU as well as the German Animal Welfare Act. The transgenic zebrafish line Tg(sox17:EGFP) [13] , [18] was used for visualizing endodermal cells during gastrulation. Embryos were collected after fertilization and incubated at 32 °C to speed up development while the temperature during imaging was kept constant at 24 °C. For morphant experiments, embryos were injected with 10 ng of cxcr4a morpholino (5′-AGACGATGTGTTCGTAATAAGCCAT-3′) at the 1-cell stage [12] . Sample embedding Low-melting agarose (1.5%) solution was prepared in E3 medium and maintained at 37 °C. At 30% epiboly stage, embryos with chorion were transferred into low-melting agarose and sucked into a cleaned FEP tube [6] (inner diameter: 2.0 mm, wall thickness: 0.5 mm), using a syringe and needle. The embryos are positioned on top of each other with minimum gap between them. The agarose was allowed to solidify at room temperature for 5 min and the FEP tube was mounted on the stage, dipping from the top into the sample chamber filled with E3 medium for time-lapse acquisition. Time-lapse acquisition The zebrafish embryo was moved along the detection axis through the alternating light sheets to acquire a z -stack of 402 planes. The two cameras were triggered simultaneously by the stage every 2 μm, acquiring one projection for each combination of illumination side and camera. The laser light was triggered when the entire chip was exposed avoiding any artefacts due to the rolling shutter. The sample was then rotated by 45° to acquire a second view, generating a total of eight projections at each time point. These steps were repeated at an interval of 30 s for a period of 12 h. In parallel, the eight projections were fused using nonlinear blending to generate a single data set based on the transformations pre-calculated with the bead sample. For imaging multiple samples in parallel, we omitted the rotation of the sample. Instead, a z -stack was acquired for one embryo and the stage translated the tube along the y axis to position the next embryo in front of the objective lenses. By repeating this, a time point is acquired for each sample and the stage moves back to bring the first embryo in the field of view. This entire process is repeated for time-lapse acquisition of multiple samples. To confirm that the laser light does not induce any developmental defects we compared two embryos that were embedded in the same tube. One was imaged for 12 h, whereas the other one was not exposed to any laser light. We found no morphological differences ( Supplementary Fig. S9 ) and both embryos were raised without defects. We also performed a timelapse with reduced speed, in which an embryo was imaged only every 15 min. We could not observe any difference to an embryo that was imaged every 30 s, as usually done in single-sample experiments ( Supplementary Movie 15 ). At the end of an experiment we captured another transmission stack to verify that the initially fitted sphere model had been valid during the course of the entire timelapse. Registration of time points When the embryonic axis forms towards the end of gastrulation, the embryo inside the chorion turns by 90°. To separate this global movement from local cell movements, images of consecutive time points were registered rigidly ( Supplementary Movies 4 and 5 ). For this purpose, the Fuller projection was calculated at each time point and smoothed using a Gaussian kernel with σ =1.5. ImageJ’s MaximumFinder plugin was used to detect local image maxima with an intensity tolerance of 10, which detected the centres of the majority of cells. The best rigid transformation between the cell centres of consecutive time points was then estimated using the Iterative Closest Point algorithm [21] , [22] . Real-time processing The software for radial projection can be applied both in real-time (images obtained directly from the camera) and post-processing (images read from the hard drive). To ensure that our software is working correctly we performed a time-lapse experiment with reduced temporal resolution, allowing us to save the raw image data. We then calculated radial projections post-processing and compared it to the raw data for consistency. Using offline data we found that our processing framework can deal with data rates of up to 250 f.p.s. Acquisition computers used for real-time processing were two Dell T7500 workstations (2 × 2.3 GHz Dual-Core, 60 GB RAM). As soon as projections were created on the acquisition computers, they are copied via a gigabit Ethernet connection to a Mac Pro workstation (2 × 2.26 GHz Quad-Core Intel Xeon, 32 GB RAM) for fusion, registration and map projections. The source code for radial maximum projection, fusion, registration and map projection is publicly available ( Supplementary Software 1 ). 2D map projections Generally, map projections aim to find a planar projection of a spherical surface such that angles, areas, distances and shapes are preserved. However, it is impossible to meet all of these requirements in a single projection, and therefore, many different types of projections have been invented. Applied to our biological data, the distortions introduced by a particular projection type influence the interpretation of the data, so that the choice for a projection needs to be taken with care. In our application we are quantifying and visualizing cellular movement of the endoderm. For analysing directionality of cell flow, the Mercator projection is ideal as it is conformal, that is, angle-preserving. To study the density of cells, area-preserving projections such as the Bonne or Gall-Peters projections are preferred. Finally, for the visualization of the global cellular flow projections reducing the overall shape distortions are preferable, such as the Fuller and Winkel Tripel projections. Map projections are ideal for visualization, as they depict the entire surface in a single 2D image. For further processing and quantification, however, we chose to use the raw vertex data where possible to avoid distortions. The final projections depict the data in polar coordinates instead of Cartesian coordinates. This way slight size differences between embryos are eliminated and their cellular pattern can be directly compared. In our projections, the commonly used scale bar is not applicable any more. The radius of the sphere provides the necessary information about the dimensions of the embryo. Distortions in the Mercator projection resulting from an incorrectly determined centre or a non-spherical embryo have been quantified ( Supplementary Fig. S10 ) and would allow us to identify and reject such data. A Java library that was originally designed for cartography and implements all common map projections ( http://www.jhlabs.com/java/maps/proj ) was used to map the spherical data on to 2D planar images. Cell segmentation and tracking The projected raw images were processed with a Retinex filter 23 to enhance the local image contrast and reduce spatial in homogeneity in image intensities. A total-variation filter was applied to reduce noise while preserving image structures 24 . Both filters were implemented in C++. Cells were detected in the Mercator projections by applying an active contours method, which allowed us to control spatial regularity of detected cell shapes 25 . An adapted size constraint was used to eliminate small, noisy artefacts, where the local area distortions of the mapping were explicitly taken into account by using an adaptive size constraint with respect to the latitude position of each cell. Each cell was tagged with an individual ID with connected component labelling. Dense deformation fields between consecutive frames were obtained by applying a fast fluid image registration 26 . Cells were finally tracked by propagating the detected cell masks with the obtained flow fields from the registration and subsequent consistency check 27 ( Supplementary Methods ). All methods were implemented in Mathematica v8.0 (Wolfram Research) except for the registration and raw segmentation (C++). Feature quantification and visualization All relevant features were evaluated either in the suitable projections or in spherical coordinates: directions of cell migration on the conformal Mercator map, densities on the area-preserving Bonne projection and distances were evaluated as great circle distances in the original spherical coordinates. Overlays of cell tracks from multiple samples were computed after alignment of all samples to the position of the DFCs at tailbud stage. Streamline plots, that is, lines of flow that are tangential to the flow vectors at each point, were computed from a static global flow field obtained by estimating the mean flow direction at each point in space. Flow directions were estimated by computing the average direction (vector sum of normalized directions) of trajectory samples (length n =10 data points) in a spatial box around each point. The margin around the DFCs was analysed by calculating the distance of each cell from the DFC and subsequent binning of the obtained distances. Radial histograms from each time point were concatenated to produce the kymographs ( Supplementary Fig. S8 ). The radii of the margin around the DFC were estimated by the 0.1 quantile of the annular distribution for each time point. The planar visualizations were computed in Mathematica, and volume renderings were done with custom Python scripts and Blender ( http://www.blender.org/ ). Analysis of movies (fluid registration, cell detection, tracking and visualization) was done on a MacBook Pro with 8GB of RAM and a QuadCore 2.3 GHz Intel Core i7. To further speedup post-processing and analysis of multi-sample data, several movies were processed in parallel on a compute server with 24 Intel Xeon CPUs running at 2.67 GHz. How to cite this article: Schmid, B. et al. High-speed panoramic light-sheet microscopy reveals global endodermal cell dynamics. Nat. Commun. 4:2207 doi: 10.1038/ncomms3207 (2013).